miR-155 regulates differentiation of brown and beige adipocytes via a bistable circuit Brown adipocytes are a primary site of energy expenditure and reside not only in classical brown adipose tissue but can also be found in white adipose tissue. Here we show that microRNA 155 is enriched in brown adipose tissue and is highly expressed in proliferating brown preadipocytes but declines after induction of differentiation. Interestingly, microRNA 155 and its target, the adipogenic transcription factor CCAAT/enhancer-binding protein β, form a bistable feedback loop integrating hormonal signals that regulate proliferation or differentiation. Inhibition of microRNA 155 enhances brown adipocyte differentiation and induces a brown adipocyte-like phenotype (‘browning’) in white adipocytes. Consequently, microRNA 155-deficient mice exhibit increased brown adipose tissue function and ‘browning’ of white fat tissue. In contrast, transgenic overexpression of microRNA 155 in mice causes a reduction of brown adipose tissue mass and impairment of brown adipose tissue function. These data demonstrate that the bistable loop involving microRNA 155 and CCAAT/enhancer-binding protein β regulates brown lineage commitment, thereby, controlling the development of brown and beige fat cells. Interscapular brown adipose tissue (BAT) is important for thermoregulation, especially during the neonatal period, but recent studies have clearly demonstrated metabolically active BAT also in adult humans [1] , [2] . Interestingly, BAT activity in adults is significantly reduced in obese subjects [3] . Brown fat-like cells have also been found within white adipose tissue (WAT) depots. The number and activity of these ‘inducible’ brown adipocytes, also known as beige or brite (BRown-in-whITE) cells, can be readily increased by cold exposure (a process also known as ‘browning’) [4] . Although activation of β-adrenergic signalling is an important stimulus for browning, not much is known about other mechanisms including microRNAs (miRNAs) that might regulate this complex process. miRNAs are small non-coding RNAs that regulate gene expression at the post-transcriptional level [5] , [6] , [7] . miRNAs are beginning to emerge as important factors that regulate differentiation of white [8] , [9] , [10] and brown fat cells [11] , [12] . Different phases of adipogenesis have been identified in both white and brown adipocytes that are tightly controlled by adipogenic transcription factors [13] . The initial phase of adipogenesis is characterized by proliferation of preadipocytes/mesenchymal stem cells followed by growth arrest induced by contact inhibition. Adipogenesis-inducing hormones promote cell cycle reentry and synchronous cell division (mitotic clonal expansion, MCE). This process is dependent on induction of two members of the CCAAT/enhancer-binding protein (C/EBP) family of transcription factors: C/EBPβ and -δ [13] . C/EBPβ activates transcription of C/EBPα and peroxisome-proliferator-activated receptor γ (PPARγ), the major transcriptional inducers of adipogenic gene expression [14] . Both PPARγ and C/EBPα are antimitotic, therefore, the timing of C/EBPβ activation is critical, because premature expression of the late transcription factors would prevent MCE [15] . Apart from its general role in adipogenesis, C/EBPβ is essential for BAT development [16] , [17] and cooperates with coregulatory protein PR domain containing 16 (PRDM16) as crucial switch in brown fat cell fate determination [18] . Furthermore, C/EBPβ is a key transcriptional inducer of uncoupling protein 1 (UCP1) expression and the thermogenic program [16] , [18] . So far, miRNA 155 (miR-155) has been mainly studied in the context of hematopoiesis, immune response and tumour formation [19] . Here we report that miR-155 constitutes a double-negative feedback loop together with its primary target C/EBPβ, thereby establishing a bistable mechanism controlling brown adipocyte differentiation and ‘browning’ of white adipocytes. miR-155 inhibits brown fat cell differentiation To identify miRNAs with a putative function in BAT differentiation, we compared miRNA expression profiles of preadipocytes isolated from the stromal vascular fraction (SVF) of BAT [20] with differentiated ( Supplementary Fig. S1a ) mature brown adipocytes by a global deep sequencing analysis. A total of 288 miRNAs could be detected in this screen: 16 miRNAs were >2-fold higher expressed in mature adipocytes differentiated in vitro , whereas 12 miRNAs were >2-fold downregulated during differentiation ( Fig. 1a ). The expression of a selected group of miRNAs was validated by quantitative real-time PCR (qRT–PCR) ( Supplementary Fig. S1b ). The three most differentially expressed miRNAs—miR-146a, miR-155 and miR-223—were analysed in more detail using lentiviral vectors carrying optimized miRNA precursor expression cassettes ( Supplementary Fig. S1c ). As a general parameter of fat cell differentiation, we analysed lipid accumulation by Oil Red O staining. Because overexpression of miR-155 (LVmiR155) dramatically reduced lipid accumulation, we focused on this miRNA in our further studies ( Supplementary Fig. S1d,e ). In addition, recent studies identified C/EBPβ as a miR-155 target gene in inflammatory processes as well as in in vitro models of white adipogenesis [19] , [21] , [22] , [23] , [24] . We found that C/EBPβ was significantly reduced in miR-155-overexpressing brown preadipocytes ( Supplementary Fig. S2a ). 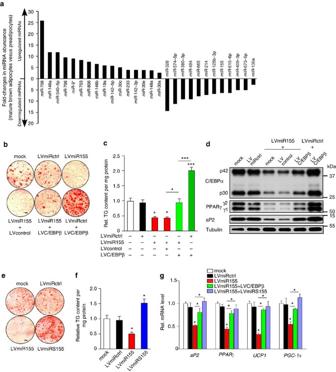Figure 1: miR-155 regulates brown fat cell differentiation via targetingC/EBPβ. (a) Genome-wide deep sequencing screen to identify differentially regulated miRNAs in brown adipocytes. The 16 upregulated and 12 downregulated miRNAs with fold changes >2 are shown. (b) Oil Red O staining ofin vitrodifferentiated brown adipocytes infected with different combinations of lentiviral vectors expressing miR-155 (LVmiR155) and/or C/EBPβ (LVC/EBPβ, 1 ng reverse transcriptase (RTase) of concentrated virus); mock, uninfected cells; LVmiRctrl, cells transduced with a control scrambled miRNA lentivirus; LVcontrol, empty vector. Scale bar, 3 mm. (c) TG content ofin vitrodifferentiated brown adipocytes transduced with combinations of lentiviral vectors expressing miR-155 (LVmiR155) and/or C/EBPβ (LVC/EBPβ, 1ng RTase); mock, uninfected cells; LVmiRctrl, cells transduced with a lentivirus carrying a scrambled miRNA; LVcontrol, empty vector; TG content was normalized to total protein concentration. Untreated control was set as one. Data are represented as means±s.e.m. (*P<0.05; ***P<0.001; one-way analysis of variance (ANOVA);n=3). (d) Western Blot analysis of fat cell markers C/EBPα, PPARγ and aP2 ofin vitrodifferentiated brown adipocytes transduced with combinations of lentiviral vectors expressing miR-155 (LVmiR155) and/or C/EBPβ (LVC/EBPβ, 1 ng RTase); mock, uninfected cells; LVmiRctrl, cells transduced with a control scrambled miRNA lentivirus; LVcontrol, empty vector. Tubulin served as loading control (representative blot out ofn=3 is shown). (e) Oil Red O staining of cells overexpressing miR-155 (LVmiR155) or an anti-miR-155 sponge (LVmiRS155) as compared with cells carrying a control scrambled miRNA (LVmiRctrl); mock, uninfected cells. Scale bar, 3 mm. (f) TG content of differentiated brown adipocytes transduced with LVmiRctrl, LVmiR155 and LVmiRS155; mock, uninfected control. TG content was normalized to total protein concentration. Untreated cells were set as one. Data are represented as means±s.e.m. (*P<0.05; one-way ANOVA;n=4). (g) Abundance of adipogenic markersaP2,PPARγ as well as of thermogenic genesUCP1andPGC-1αas measured by qRT–PCR. Untreated cells (mock) were set as one; data are presented as means±s.e.m. (*P<0.05; one-way ANOVA;n=3). Figure 1: miR-155 regulates brown fat cell differentiation via targeting C/EBPβ. ( a ) Genome-wide deep sequencing screen to identify differentially regulated miRNAs in brown adipocytes. The 16 upregulated and 12 downregulated miRNAs with fold changes >2 are shown. ( b ) Oil Red O staining of in vitro differentiated brown adipocytes infected with different combinations of lentiviral vectors expressing miR-155 (LVmiR155) and/or C/EBPβ (LVC/EBPβ, 1 ng reverse transcriptase (RTase) of concentrated virus); mock, uninfected cells; LVmiRctrl, cells transduced with a control scrambled miRNA lentivirus; LVcontrol, empty vector. Scale bar, 3 mm. ( c ) TG content of in vitro differentiated brown adipocytes transduced with combinations of lentiviral vectors expressing miR-155 (LVmiR155) and/or C/EBPβ (LVC/EBPβ, 1ng RTase); mock, uninfected cells; LVmiRctrl, cells transduced with a lentivirus carrying a scrambled miRNA; LVcontrol, empty vector; TG content was normalized to total protein concentration. Untreated control was set as one. Data are represented as means±s.e.m. (* P <0.05; *** P <0.001; one-way analysis of variance (ANOVA); n =3). ( d ) Western Blot analysis of fat cell markers C/EBPα, PPARγ and aP2 of in vitro differentiated brown adipocytes transduced with combinations of lentiviral vectors expressing miR-155 (LVmiR155) and/or C/EBPβ (LVC/EBPβ, 1 ng RTase); mock, uninfected cells; LVmiRctrl, cells transduced with a control scrambled miRNA lentivirus; LVcontrol, empty vector. Tubulin served as loading control (representative blot out of n =3 is shown). ( e ) Oil Red O staining of cells overexpressing miR-155 (LVmiR155) or an anti-miR-155 sponge (LVmiRS155) as compared with cells carrying a control scrambled miRNA (LVmiRctrl); mock, uninfected cells. Scale bar, 3 mm. ( f ) TG content of differentiated brown adipocytes transduced with LVmiRctrl, LVmiR155 and LVmiRS155; mock, uninfected control. TG content was normalized to total protein concentration. Untreated cells were set as one. Data are represented as means±s.e.m. (* P <0.05; one-way ANOVA; n =4). ( g ) Abundance of adipogenic markers aP2 , PPAR γ as well as of thermogenic genes UCP1 and PGC-1α as measured by qRT–PCR. Untreated cells (mock) were set as one; data are presented as means±s.e.m. (* P <0.05; one-way ANOVA; n =3). Full size image For C/EBPβ, three different polypeptides are generated: two activating forms termed LAP and LAP* (liver-enriched transcriptional activator protein) and one inhibitory form named LIP (liver-enriched transcriptional inhibitory protein) [25] . The three isoforms arise from one single mRNA transcript with the same 3′ untranslated region (UTR) containing the miR-155 recognition site due to alternative translation initiation sites [26] . We found that miR-155 downregulates all three C/EBPβ isoforms ( Supplementary Fig. S2b ). In our analyses, we were focusing on the LAP isoforms, because these are the predominant ones in brown adipocytes and have been shown to bind to PRDM16 [18] . Databases are currently annotating more than 250 conserved miR-155 target genes ( www.targetscan.org ). Using luciferase constructs, we verified a direct interaction of miR-155 with C/EBPβ in brown preadipocytes ( Supplementary Fig. S2c ). Importantly, restoration of physiological C/EBPβ expression levels with a lentiviral vector carrying a C/EBPβ cDNA that lacks the miR-155 3′ UTR target sequence (LVC/EBPβ) ( Supplementary Fig. S2d ) rescued the effect of miR-155 on lipid accumulation ( Fig. 1b ). In addition, transduction with LVC/EBPβ restored expression of the adipogenic markers C/EBPα, PPARγ and fatty-acid-binding protein 4 (aP2) ( Fig. 1d ). Next, we investigated the effects of endogenous miR-155 on adipogenesis by a lentiviral vector carrying a miR-155-specifc octameric decoy target (LVmiRS155)—a so called ‘sponge’ [27] —that competitively inhibits miR-155 ( Supplementary Fig. S1c,d ). miR-155 inhibition with the sponge construct resulted in higher abundance of C/EBPβ and clearly increased luciferase reporter activity ( Supplementary Fig. S2e,f ). In addition, LVmiRS155-transduced cells displayed a significant increase in lipid droplet content and triglyceride (TG) ( Fig. 1e ). Western blotting revealed that expression of the miR-155 sponge effectively increased the abundance of C/EBPα, PPARγ and aP2 as compared with wild-type (wt) cells or LVmiRctrl-transduced cells ( Supplementary Fig. S2g,h ). Because the thermogenic program of BAT cells can be regulated independently of adipogenic differentiation [28] , we measured expression of PPARγ-coactivator 1α ( PGC-1α ), a key regulator of mitochondrial biogenesis and oxidative metabolism [29] , and UCP1 [30] , which disrupts the mitochondrial proton gradient leading to dissipation of energy as heat. The reduction of UCP1 and PGC-1α in miR-155-overexpressing cells was restored by LVC/EBPβ ( Fig. 1g ). In addition, inactivation of miR-155 significantly increased expression of thermogenic markers in wt as well as in LVmiR155 transduced cells ( Fig. 1g and Supplementary Fig. S2i ). Thus, miR-155 efficiently inhibits adipogenic differentiation and development of the thermogenic program in brown adipocytes. miR-155 is induced by transforming growth factor-β1 in preadipocytes Analysis of miR-155 expression during BAT differentiation revealed that miR-155 expression peaks when cells reach confluency around day −1 of the differentiation protocol ( Supplementary Fig. S1a ) and decreases continuously after induction of adipogenesis ( Fig. 2a ). Transforming growth factor-β1 (TGFβ1) increases miR-155 in epithelial cells [31] . Furthermore, TGFβ1 has been shown to potently inhibit adipogenesis in 3T3-L1 cells [32] . Therefore, we addressed the question if TGFβ1/Smad signalling is regulating miR-155 expression in brown fat cells. Treatment of preadipocytes with TGFβ1 significantly increased miR-155 levels within 24 h ( Fig. 2b ), whereas inhibition of Smad4 blocked TGFβ1-mediated miR-155 induction ( Supplementary Fig. S3a,b ). Interestingly, we found that TGFβ1 is expressed by brown preadipocytes and is regulated in a differentiation-dependent manner similar to miR-155 ( Fig. 2a ). 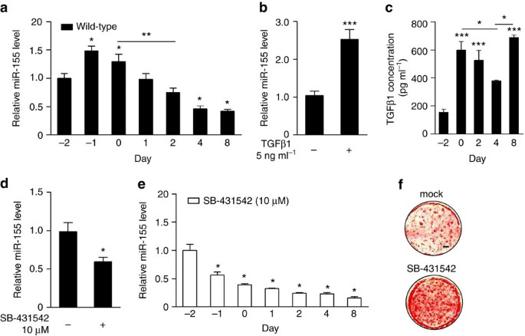Figure 2: miR-155 expression is induced by TGFβ signalling during brown cell differentiation. (a) qRT–PCR analysis of miR-155 expression levels in brown fat cells duringin vitrodifferentiation (normalized to snoRNA202). Undifferentiated cells (day 2) were set as one. Data are represented as means±s.e.m. (*P<0.05; **P<0.005; one-way analysis of variance (ANOVA);n=5). (b) Effect of TGFβ1 (5 ng ml−1, 24 h) on miR-155 expression in brown fat cells as measured by qRT–PCR (normalized to snoRNA202 expression). Untreated cells were set as one. Data are represented as means±s.e.m. (***P<0.001; Student’st-test;n=3). (c) TGFβ1 concentration in the cell culture supernatant during brown fat cell differentiation. Data are represented as means±s.e.m. (*P<0.05; ***P<0.001; one-way ANOVA;n=3). (d) Effect of SB-431542 (10 μM, 24 h) on miR-155 expression as measured by qRT–PCR (normalized to snoRNA202). Data are represented as means±s.e.m. (*P<0.05; Student’st-test, as compared with untreated controls;n=3). (e) qRT–PCR analysis of miR-155 expression inin vitrodifferentiated brown fat cells treated with SB-431542 (10 μM, treatment day −2 to day 0) (normalized to snoRNA202). Undifferentiated cells (day −2) were set as one. Data are represented as means±s.e.m. (*P<0.05; one-way ANOVA;n=3) (f) Oil Red O staining ofin vitrodifferentiated brown adipocytes treated with SB-431542 (10 μM, day −2 to day 0); mock, untreated cells. Scale bar, 3 mm. Figure 2: miR-155 expression is induced by TGFβ signalling during brown cell differentiation. ( a ) qRT–PCR analysis of miR-155 expression levels in brown fat cells during in vitro differentiation (normalized to snoRNA202). Undifferentiated cells (day 2) were set as one. Data are represented as means±s.e.m. (* P <0.05; ** P <0.005; one-way analysis of variance (ANOVA); n =5). ( b ) Effect of TGFβ1 (5 ng ml −1 , 24 h) on miR-155 expression in brown fat cells as measured by qRT–PCR (normalized to snoRNA202 expression). Untreated cells were set as one. Data are represented as means±s.e.m. (*** P <0.001; Student’s t -test; n =3). ( c ) TGFβ1 concentration in the cell culture supernatant during brown fat cell differentiation. Data are represented as means±s.e.m. (* P <0.05; *** P <0.001; one-way ANOVA; n =3). ( d ) Effect of SB-431542 (10 μM, 24 h) on miR-155 expression as measured by qRT–PCR (normalized to snoRNA202). Data are represented as means±s.e.m. (* P <0.05; Student’s t -test, as compared with untreated controls; n =3). ( e ) qRT–PCR analysis of miR-155 expression in in vitro differentiated brown fat cells treated with SB-431542 (10 μM, treatment day −2 to day 0) (normalized to snoRNA202). Undifferentiated cells (day −2) were set as one. Data are represented as means±s.e.m. (* P <0.05; one-way ANOVA; n =3) ( f ) Oil Red O staining of in vitro differentiated brown adipocytes treated with SB-431542 (10 μM, day −2 to day 0); mock, untreated cells. Scale bar, 3 mm. Full size image Furthermore, inhibition of TGFβ1 signalling with SB-431542 (ref. 33 ) clearly reduced miR-155 levels ( Fig. 2d ). Interestingly, SB-431542 treatment resulted in enhanced adipogenesis ( Fig. 2f ). The most prominent effects of SB-431542 on differentiation were observed between day −4 to day 0 ( Supplementary Fig. S3c ), which correlates with the time point of TGFβ1-mediated induction of miR-155. These pro-adipogenic effects of inhibition of TGFβ signalling were clearly abolished in LVmiR155-expressing cells, indicating that miR-155 is a crucial downstream effector of TGFβ signalling in brown adipogenesis ( Supplementary Fig. S3d ). miR-155 and C/EBPβ form a bistable loop To identify mechanisms that—apart from TGFβ1—might regulate miR-155, we examined the miR-155 promoter sequence for transcription-factor-binding sites. miR-155 is processed from a primary transcript, the B-cell integration cluster (BIC) [34] , [35] . Analysis of the BIC/miR-155 promoter sequence revealed putative C/EBP-binding motifs ( Fig. 3a ) indicating that miR-155 might be regulated by its own target through a feedback mechanism. C/EBPβ is tightly regulated during fat cell differentiation: expression is almost undetectable in preadipocytes and is strongly induced by the adipogenic cocktail applied at day 0 ( Fig. 3b ), the time point when miR-155 expression is beginning to decrease. Overexpression of C/EBPβ in brown preadipocytes caused a dramatic downregulation of miR-155 levels ( Fig. 3d ). Next, we used BIC/miR-155 promoter reporter constructs, to analyse transcriptional regulation of miR-155 by C/EBPβ in more detail. Overexpression of C/EBPβ led to a pronounced inhibition of BIC/miR-155 promoter activity in HIB-1B brown preadipocytes ( Fig. 3e ). In contrast, siRNA-mediated knockdown of C/EBPβ (siC/EBPβ) caused a significant increase in miR-155 expression in BAT-derived preadipocytes ( Supplementary Fig. S4a,b ). 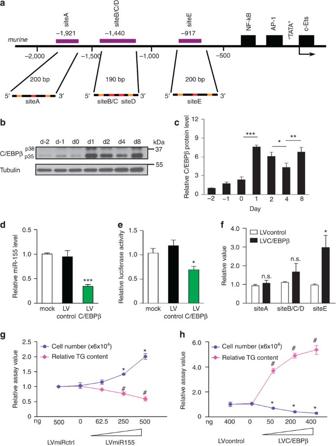Figure 3: miR-155 and C/EBPβ constitute a bistable feedback loop. (a) Scheme of the 2 kb murine BIC/miR-155 promoter with the putative C/EBP-binding sites (siteA, siteB/C/D and siteE) (purple); primer binding sites, orange; C/EBP binding sites, red. (b) Representative western blot of C/EBPβ expression duringin vitrobrown fat differentiation. Protein samples were collected at indicated time points. Tubulin served as loading control. (c) Densitometric analysis of C/EBPβ protein levels normalized to tubulin. Data from day −2 were set as one; all data are represented as means±s.e.m. (*P<0.05; **P<0.01; ***P<0.001; one-way analysis of variance (ANOVA);n=3). (d) qRT–PCR analysis of miR-155 expression (normalized to sno202) in cells transduced with LVC/EBPβ or control virus (LVcontrol). Untreated controls (mock) were set as one; data are represented as means±s.e.m. (***P<0.001; one-way ANOVA;n=3). (e) Luciferase assay to analyse regulation of the BIC/miR-155 promoter by C/EBPβ. Cells were infected with LVcontrol or LVC/EBPβ 48 h before BIC/miR-155 promoter luciferase construct transfection. Uninfected controls (mock), transfected with the same reporter construct were set as one; data are represented as means±s.e.m. (*P<0.05; one-way ANOVA;n=4). (f) Brown preadipocytes were transduced with LVcontrol or LVC/EBPβ 48 h prior the Chromatin immunoprecipitation assay. Precipitation was performed with an anti-C/EBPβ antibody or IgG and PolII control antibodies. C/EBPβ-bound BIC/miR-155 promoter fragments were amplified using qRT–PCR primers that span putative binding sites A, B/C/D or E, respectively. Results are normalized to input values. Relative values are represented as means±s.e.m. (*P<0.05; Student’st-test; n.s., not significant;n=3). (g,h) TG content and cell number of brown adipocytes transduced with different doses of (g) LVmiR155 (0, 62.5, 250 and 500 ng RTase per well in six-well plates) or (h) LVC/EBPβ (0, 50, 200 and 400 ng RTase per well in six-well plates). TG content was normalized to total protein concentration. LVmiRctrl-transduced cells were set as one. All data are represented as means±s.e.m. (#P<0.05; one-way ANOVA;n=3 in TG assay, *P<0.05; one-way ANOVA;n=3 in proliferation assay). Figure 3: miR-155 and C/EBPβ constitute a bistable feedback loop. ( a ) Scheme of the 2 kb murine BIC/miR-155 promoter with the putative C/EBP-binding sites (siteA, siteB/C/D and siteE) (purple); primer binding sites, orange; C/EBP binding sites, red. ( b ) Representative western blot of C/EBPβ expression during in vitro brown fat differentiation. Protein samples were collected at indicated time points. Tubulin served as loading control. ( c ) Densitometric analysis of C/EBPβ protein levels normalized to tubulin. Data from day −2 were set as one; all data are represented as means±s.e.m. (* P <0.05; ** P <0.01; *** P <0.001; one-way analysis of variance (ANOVA); n =3). ( d ) qRT–PCR analysis of miR-155 expression (normalized to sno202) in cells transduced with LVC/EBPβ or control virus (LVcontrol). Untreated controls (mock) were set as one; data are represented as means±s.e.m. (*** P <0.001; one-way ANOVA; n =3). ( e ) Luciferase assay to analyse regulation of the BIC/miR-155 promoter by C/EBPβ. Cells were infected with LVcontrol or LVC/EBPβ 48 h before BIC/miR-155 promoter luciferase construct transfection. Uninfected controls (mock), transfected with the same reporter construct were set as one; data are represented as means±s.e.m. (* P <0.05; one-way ANOVA; n =4). ( f ) Brown preadipocytes were transduced with LVcontrol or LVC/EBPβ 48 h prior the Chromatin immunoprecipitation assay. Precipitation was performed with an anti-C/EBPβ antibody or IgG and PolII control antibodies. C/EBPβ-bound BIC/miR-155 promoter fragments were amplified using qRT–PCR primers that span putative binding sites A, B/C/D or E, respectively. Results are normalized to input values. Relative values are represented as means±s.e.m. (* P <0.05; Student’s t -test; n.s., not significant; n =3). ( g , h ) TG content and cell number of brown adipocytes transduced with different doses of ( g ) LVmiR155 (0, 62.5, 250 and 500 ng RTase per well in six-well plates) or ( h ) LVC/EBPβ (0, 50, 200 and 400 ng RTase per well in six-well plates). TG content was normalized to total protein concentration. LVmiRctrl-transduced cells were set as one. All data are represented as means±s.e.m. ( # P <0.05; one-way ANOVA; n =3 in TG assay, * P <0.05; one-way ANOVA; n =3 in proliferation assay). Full size image Because the motifs in the BIC/miR-155 promoter region ( Fig. 3a ) are predicted to be generally targeted by C/EBPs, we directly compared the effects of C/EBPα, β and δ on BIC/miR-155 promoter activity. All members of the C/EBP transcription factor family can contribute to suppression of miR-155 during later stages of differentiation ( Supplementary Fig. S4c ). Importantly, C/EBPβ is the only C/EBP family member that contains miR-155 binding sites in its 3′ UTR ( www.targetscan.org ). Therefore, the newly described feedback loop is strictly limited to miR-155 and C/EBPβ. Chromatin immunoprecipitation assays identified the distal siteE in the BIC/miR-155 promoter as the critical binding site for C/EBPβ ( Fig. 3f ). These data indicate that miR-155 and its target C/EBPβ constitute a double-negative feedback loop in brown preadipocytes. Such feedback loops are important in developmental transcriptional regulation and are known to exhibit a bistable behaviour [36] . To analyse whether miR-155 and C/EBPβ regulate each other in a direct, dose-dependent manner, preadipocytes were infected with increasing amounts of lentiviruses either expressing miR-155 or C/EBPβ ( Supplementary Fig. S4d–g ). Stepwise increase in miR-155 levels ( Supplementary Fig. S4d ) resulted in a dose-dependent reduction of C/EBPβ ( Supplementary Fig. S4e ). On the other hand, increasing the abundance of C/EBPβ to levels observed after induction of brown fat differentiation resulted in a dose-dependent reduction of miR-155 ( Supplementary Fig. S4f,g ). To better understand the relevance of this reciprocal inhibition, we analysed the influence of miR-155 and C/EBPβ on the differentiation state of brown fat cells. miR-155 overexpression correlated with decreased cellular TG content and enhanced proliferation ( Fig. 3g ). In contrast, C/EBPβ overexpression had the opposite effects resulting in strongly increased TG levels and significant reduction of proliferation ( Fig. 3h ). Preadipocyte factor 1 (Pref-1), a transmembrane protein highly expressed in undifferentiated preadipocytes [37] , was highly expressed in miR-155-overexpressing cells ( Supplementary Fig. S4h,i ). In contrast, cells with low miR-155 ( Supplementary Fig. S4h ) or high C/EBPβ levels ( Supplementary Fig. S4j ) displayed strongly reduced Pref-1 expression. These data indicate that miR-155 and C/EBPβ constitute a bistable system/loop that either maintains preadipocytes in a proliferative, undifferentiated stem cell state or initiates the brown adipogenic differentiation. miR-155 suppresses brown adipogenesis in vivo Next, we analysed miR-155 expression in different fat depots. We found significantly higher levels of miR-155 in BAT compared with inguinal WAT (igWAT) ( Fig. 4a ). Similar to the in vitro situation, we found high levels of miR-155 in the SVF as well as in the purified (Sca1 + /CD45 − /Mac1 − ) precursors, whereas mature brown adipocytes exhibited a 2.6-fold reduction of miR-155 ( Supplementary Fig. S5a,b ). 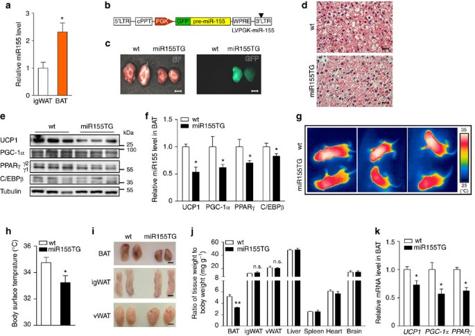Figure 4: miR-155 impairs brown fat differentiationin vivo. (a) qRT–PCR analysis for miR-155 expression in igWAT and BAT of 10-week-old male mice. Expression in igWAT was set as one;n=3. (b) Schematic representation of the lentiviral construct (LVPGK-miR-155) used for generation of miR-155 transgenic (miR155TG) animals. For abbreviations, seeSupplementary Fig. S1, PGK, phosphoglycerate 1 promoter. (c) Interscapular BAT isolated from 1-week-old wt or miR155TG mice. Bright field (left) and fluorescent images (right) are shown; GFP is co-expressed with miR-155 in transgenic mice; (scale bar =2 mm). (d) Hematoxylin and eosin staining of BAT sections from 1-week-old wt and miR155TG littermates; (scale bar =15 μm). (e) Western blot analysis of UCP1, PGC-1α, PPARγ and C/EBPβ expression in BAT isolated from 1-week-old wt and miR155TG littermates; each protein levels from three representative animals per group are shown. Tubulin served as loading control. (f) Densitometric quantification of UCP1, PGC-1α, PPARγ and C/EBPβ expression levels, normalized to tubulin. Data of the wt group were set as one;n=6 per group. (g) Infrared thermographic analysis of the body surface temperature in 4-day-old wt and miR155TG littermates. Three representative pairs are showed. (h) Statistical analysis of body surface temperature in wt and miR155TG littermates; wt: 34.75±0.39 °C; miR155TG: 33.24±0.53 °C;n=5 per group. (i) Interscapular BAT, igWAT, and visceral WAT (vWAT) were isolated from 10-week-old wt or miR155TG littermates. Scale bar, 3 mm (BAT); 4 mm (igWAT and vWAT). Two representative littermates are shown. (j) Statistics of BAT, igWAT, vWAT, spleen, heart, brain and liver weights relative to total body weight in 10-week-old wt and miR155TG littermates;n=3 per group. (k) qRT–PCR analysis of brown thermogenic/adipogenic genes in interscapular BAT of wt or miR155TG littermates at 10 weeks of age:UCP1,PGC-1αandPPARγ;n=3 per group. All data are presented as means±s.e.m. (*P<0.05; **P<0.01; n.s., not significant; Student’st-test). Figure 4: miR-155 impairs brown fat differentiation in vivo. ( a ) qRT–PCR analysis for miR-155 expression in igWAT and BAT of 10-week-old male mice. Expression in igWAT was set as one; n =3. ( b ) Schematic representation of the lentiviral construct (LVPGK-miR-155) used for generation of miR-155 transgenic (miR155TG) animals. For abbreviations, see Supplementary Fig. S1 , PGK, phosphoglycerate 1 promoter. ( c ) Interscapular BAT isolated from 1-week-old wt or miR155TG mice. Bright field (left) and fluorescent images (right) are shown; GFP is co-expressed with miR-155 in transgenic mice; (scale bar =2 mm). ( d ) Hematoxylin and eosin staining of BAT sections from 1-week-old wt and miR155TG littermates; (scale bar =15 μm). ( e ) Western blot analysis of UCP1, PGC-1α, PPARγ and C/EBPβ expression in BAT isolated from 1-week-old wt and miR155TG littermates; each protein levels from three representative animals per group are shown. Tubulin served as loading control. ( f ) Densitometric quantification of UCP1, PGC-1α, PPARγ and C/EBPβ expression levels, normalized to tubulin. Data of the wt group were set as one; n =6 per group. ( g ) Infrared thermographic analysis of the body surface temperature in 4-day-old wt and miR155TG littermates. Three representative pairs are showed. ( h ) Statistical analysis of body surface temperature in wt and miR155TG littermates; wt: 34.75±0.39 °C; miR155TG: 33.24±0.53 °C; n =5 per group. ( i ) Interscapular BAT, igWAT, and visceral WAT (vWAT) were isolated from 10-week-old wt or miR155TG littermates. Scale bar, 3 mm (BAT); 4 mm (igWAT and vWAT). Two representative littermates are shown. ( j ) Statistics of BAT, igWAT, vWAT, spleen, heart, brain and liver weights relative to total body weight in 10-week-old wt and miR155TG littermates; n =3 per group. ( k ) qRT–PCR analysis of brown thermogenic/adipogenic genes in interscapular BAT of wt or miR155TG littermates at 10 weeks of age: UCP1 , PGC-1α and PPARγ ; n =3 per group. All data are presented as means±s.e.m. (* P <0.05; ** P <0.01; n.s., not significant; Student’s t -test). Full size image To study the function of miR-155 in vivo , we generated transgenic mice overexpressing miR-155 under control of the ubiquitous phosphoglycerate kinase ( PGK ) promoter (miR155TG) ( Fig. 4b and Supplementary Fig. S5c ) using lentiviral transgenesis [38] , [39] . One-week-old miR155TG animals displayed significantly reduced size and weight of BAT compared with their wt littermates ( Fig. 4c and Supplementary Fig. S5d ). Similar to the in vitro situation, the size and number of lipid droplets in interscapular BAT of miR155TG ( Fig. 4d ) and TG content ( Supplementary Fig. S5e ), as well as key adipogenic and thermogenic factors ( Fig. 4e ), were clearly reduced. Remarkably, miR155TG mice displayed a significant reduction of BAT-derived thermogenesis as measured by infrared thermography [20] , [40] ( Fig. 4g ). Also at 10 weeks of age, miR155TG mice exhibited a significantly reduced interscapular BAT mass and clearly lower levels of thermogenic markers in BAT ( Fig. 4i–k ). In contrast, size and weight of igWAT and visceral WAT (vWAT) were not affected by miR-155 overexpression ( Fig. 4i ), albeit similar levels of miR-155 expression were reached in WAT and BAT ( Supplementary Fig. S5f,g ). miR155TG animals do not show significant alterations in body weight or food intake ( Supplementary Fig. S5h,i ). These data indicate a preferential effect of miR-155 on BAT development, which is reminiscent of the alterations observed in C/EBPβ-deficient mice [16] . To study whether the observed phenotype in BAT is cell autonomous, we generated an additional, BAT-specific mouse model using the UCP1 promoter to drive miR-155 expression (LVUCP1-miR-155) ( Supplementary Fig. S6a ). Transduction of brown preadipocytes with LVUCP1-miR-155 clearly reduced differentiation, demonstrating the functionality of the UCP1-miR-155 construct in brown fat cells ( Supplementary Fig. S6b ). One-week-old LVUCP1-miR-155 transgenic (LVUCP1miR155TG) animals ( Supplementary Fig. S6c ), showed a phenotype very similar to the miR155TG mice with ubiquitous miR-155 expression: Body surface temperature and BAT weight were significantly decreased ( Supplementary Fig. S6d,e ). In addition, size and number of lipid droplets in BAT ( Supplementary Fig. S6f ), as well as expression of PPARγ and UCP1, were clearly reduced ( Supplementary Fig. S6g,h ). Thus, both transgenic animal models demonstrate that miR-155 overexpression in vivo impairs BAT function. miR-155 regulates white fat browning in vitro To assess the effects of miR-155 on white fat cells, we isolated SVF cells from murine igWAT ( Supplementary Fig. S7a ) and overexpressed miR-155 using three different concentrations of LVmiR155 (60, 180 and 500 ng RTase). In addition, we knocked down miR-155 and C/EBPβ. Overexpression of miR-155 at high levels (500 ng RTase) significantly reduced lipid content ( Fig. 5a and Supplementary Fig. S7b ) and adipogenic marker levels in white adipocytes ( Fig. 5c ), whereas transduction with LVmiRS155 resulted in enhanced differentiation ( Fig. 5b ). Given the prominent effect of miR-155 on the development of the thermogenic program in brown adipocytes ( Fig. 1g ), we examined whether miR-155 might also have similar effects in WAT progenitors. Importantly, inhibition of endogenous miR-155 dramatically induced expression of UCP1 more than 20-fold ( Fig. 5d and Supplementary Fig. S7c ). Remarkably, the increase in UCP1 expression induced by the miR-155 sponge was even higher than the effect of norepinephrine, a well-known inducer of ‘browning’ [4] , and was identical to the effect of C/EBPβ overexpression ( Fig. 5d ). Although PGC-1α and Cidea were almost undetectable in WAT, both were significantly increased by knockdown of miR-155 ( Fig. 5d ). In contrast, transduction with LVmiR155 further decreased the already low expression levels of UCP1 ( Fig. 5d ). 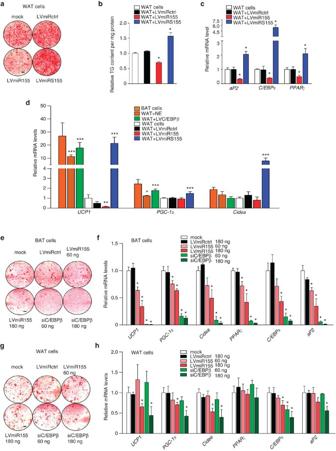Figure 5: miR-155 regulates the recruitment of brite fat cells. (a) Oil Red O staining of fully differentiated WATs overexpressing miR-155 (LVmiR155) or an anti-miR-155 sponge (LVmiRS155) as compared with cells carrying a control scrambled miRNA (LVmiRctrl); mock, uninfected cells. (b) TG content of fully differentiated white adipocytes transduced with LVmiRctrl, LVmiR155 and LVmiRS155; mock, uninfected control. TG content was normalized to total protein concentration. Untreated cells were set as one. Data are represented as means±s.e.m. (*P<0.05; one-way analysis of variance (ANOVA);n=3). (c) qRT–PCR analysis ofaP2, C/EBPαandPPARγmRNA in fully differentiated white adipocytes transduced with indicated lentiviruses. Untreated cells were set as one. Data are presented as mean±s.e.m. (*P<0.05; one-way ANOVA;n=3). (d) qRT–PCR analysis ofUCP1,PGC-1αandCideamRNA levels in differentiated white adipocytes transduced with LVC/EBPβ, LVmiR155, LVmiRS155 and LVmiRctrl or treated with 5 μM norepinephrine (NE). Differentiated BAT cells were used as positive control. Untreated white fat cells were set as one. Data were normalized toHPRThousekeeping gene expression and are represented as means±s.e.m. (*P<0.05; **P<0.01; ***P<0.001; one-way ANOVA;n=3). (e,f) Oil Red O staining (e) and qRT–PCR analysis (f) ofUCP1, PGC-1α, Cidea,PPARγ,C/EBPαandaP2mRNA of brown adipocytes (BAT cells) transduced with a low (60 ng RTase) or medium (180 ng RTase) dosage of control-miR (LVmiRctrl), miR-155 (LVmiR155) or anti-C/EBPβ siRNA (siC/EBPβ); mock, uninfected cells. Uninfected cells were set as one. Expression data are normalized toHPRT, and data are represented as means± s.e.m. (*P<0.05; one-way ANOVA;n=3). (g,h) Oil Red O staining (g) and qRT–PCR analysis (h) ofUCP1, PGC-1α, Cidea,PPARγ,C/EBPαandaP2mRNA of white adipocytes (WAT cells) transduced with with a low (60 ng RTase) or medium (180 ng RTase) dosage of control-miR (LVmiRctrl), miR-155 (LVmiR155) or anti-C/EBPβ siRNA (siC/EBPβ); mock, uninfected cells. Uninfected cells were set as one. Expression data are normalized toHPRT, and data are represented as means± s.e.m. (*P<0.05; one-way ANOVA;n=3). Scale bar, 3 mm. Figure 5: miR-155 regulates the recruitment of brite fat cells. ( a ) Oil Red O staining of fully differentiated WATs overexpressing miR-155 (LVmiR155) or an anti-miR-155 sponge (LVmiRS155) as compared with cells carrying a control scrambled miRNA (LVmiRctrl); mock, uninfected cells. ( b ) TG content of fully differentiated white adipocytes transduced with LVmiRctrl, LVmiR155 and LVmiRS155; mock, uninfected control. TG content was normalized to total protein concentration. Untreated cells were set as one. Data are represented as means±s.e.m. (* P <0.05; one-way analysis of variance (ANOVA); n =3). ( c ) qRT–PCR analysis of aP2, C/EBPα and PPARγ mRNA in fully differentiated white adipocytes transduced with indicated lentiviruses. Untreated cells were set as one. Data are presented as mean±s.e.m. (* P <0.05; one-way ANOVA; n =3). ( d ) qRT–PCR analysis of UCP1 , PGC-1α and Cidea mRNA levels in differentiated white adipocytes transduced with LVC/EBPβ, LVmiR155, LVmiRS155 and LVmiRctrl or treated with 5 μM norepinephrine (NE). Differentiated BAT cells were used as positive control. Untreated white fat cells were set as one. Data were normalized to HPRT housekeeping gene expression and are represented as means±s.e.m. (* P <0.05; ** P <0.01; *** P <0.001; one-way ANOVA; n =3). ( e , f ) Oil Red O staining ( e ) and qRT–PCR analysis ( f ) of UCP1, PGC-1α, Cidea , PPARγ , C/EBPα and aP2 mRNA of brown adipocytes (BAT cells) transduced with a low (60 ng RTase) or medium (180 ng RTase) dosage of control-miR (LVmiRctrl), miR-155 (LVmiR155) or anti-C/EBPβ siRNA (siC/EBPβ); mock, uninfected cells. Uninfected cells were set as one. Expression data are normalized to HPRT , and data are represented as means± s.e.m. (* P <0.05; one-way ANOVA; n =3). ( g , h ) Oil Red O staining ( g ) and qRT–PCR analysis ( h ) of UCP1, PGC-1α, Cidea , PPARγ , C/EBPα and aP2 mRNA of white adipocytes (WAT cells) transduced with with a low (60 ng RTase) or medium (180 ng RTase) dosage of control-miR (LVmiRctrl), miR-155 (LVmiR155) or anti-C/EBPβ siRNA (siC/EBPβ); mock, uninfected cells. Uninfected cells were set as one. Expression data are normalized to HPRT , and data are represented as means± s.e.m. (* P <0.05; one-way ANOVA; n =3). Scale bar, 3 mm. Full size image Next, we performed transduction experiments also at low and medium doses of LVmiR155 and LVsiC/EBPβ in BAT and WAT-derived adipocytes ( Fig. 5e–h ). In brown fat cells, we found a significant inhibition of differentiation already at the low dose (60 ng RTase) of miR-155 with a 28% decrease in expression of PPARγ and reduced Oil Red O staining. The thermogenic program (as determined by measurement of UCP1 and PGC-1α levels) was also significantly suppressed by low levels of miR-155 ( Fig. 5e ). In contrast, the low concentration of miR-155 had no significant effect on any of the marker genes tested during white fat cell differentiation ( Fig. 5g ). In accordance, knockdown of C/EBPβ had a more striking impact on marker expression in brown versus white fat cells ( Fig. 5e–h ). The medium dose (180 ng RTase) of miR-155 caused a significant reduction of the thermogenic marker gene expression, but was still not sufficient to significantly affect all adipogenic markers in white fat cells. siC/EBPβ significantly inhibited white adipocyte differentiation at medium concentrations (maximum suppression 55.6–60.1% at 180 ng) ( Fig. 5h ). The effects of medium-dose siC/EBPβ were much more pronounced in brown fat cells resulting in a 87.1–99.3% reduction of marker gene expression ( Fig. 5f ). All these data point towards higher sensitivity of brown adipocytes for miR-155- and C/EBPβ-dependent regulation. Analysis of miR-155-deficient mice To analyse the effect of miR-155 suppression on WAT browning and BAT recruitment in vivo , we used BIC /miR-155 -knockout (miR-155 −/− ) mice [41] . BAT activation was studied by exposing mice to cold (4 °C). Interscapular temperature of miR-155 −/− mice was significantly higher (38.4±0.66 °C) as compared with the wt littermates (35±0.37 °C) after cold exposure, indicating that inducible thermogenesis of BAT is significantly increased in the absence of miR-155 ( Fig. 6a ). In addition, analysis of body core temperature revealed a significant difference between miR-155 −/− and wt mice already at room temperature (RT). After 4 h cold exposure, core temperature dropped by 3±0.39 °C in wt but only 0.8±0.3 °C in miR-155 −/− mice ( Supplementary Fig. S8f ). 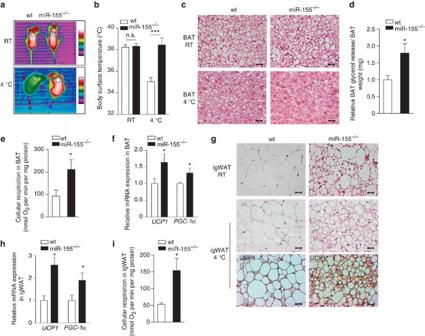Figure 6: miR-155 regulates cold-induced thermogenesis in BAT and ‘browning’ of WAT. (a) Representative infrared thermographic image of 12–16-week-old male wt and miR-155−/−littermates kept at 4 °C for 4 h. (b) Statistical analysis of body surface temperature as measured by infrared thermography. Data are represented as means±s.e.m. (***P<0.001; Student’st-test; n.s., not significant; wt groupn=7, miR-155−/−groupn=5). (c) Hematoxylin and eosin staining of interscapular BAT sections from wt and miR-155−/−littermates kept at room tempertaure (RT) or post cold exposure (4 °C, 4 h). Scale bar, 50 μm. (d) Lipolysis assay of BAT from 12-week-old wt and miR-155−/−littermates kept in 4 °C for 4 h. Data are represented as means±s.e.m. (*P<0.05; Student’st-test;n=4). (e)Ex vivooxygraph measurement of cellular mitochondrial respiration in BAT 12–16-weeks-old wt or miR-155−/−littermates exposed to 4 °C. Data are represented as means±s.e.m. (*P<0.05; Student’st-test; wt groupn=6, miR-155−/−groupn=5). (f) qRT–PCR analyses ofUCP1andPGC-1αexpression in BAT of 12–16-week-old wt or miR-155−/−littermates after cold exposure. Data are represented as means±s.e.m. (*P<0.05; Student’st-test;n=4). (g) Representative hematoxylin and eosin staining of igWAT sections from wt and miR-155−/−littermates at RT or post cold exposure (top). Immunohistochemical staining for UCP1 abundance in respective igWAT sections (bottom). Scale bar, 50 μm. (h) qRT–PCR analyses ofUCP1andPGC-1αin igWAT 12–16-week-old wt or miR-155−/−littermates exposed to 4 °C for 4 h. Data are represented as means±s.e.m. (*P<0.05; Student’st-test; wt groupn=4, miR-155−/−groupn=4). (i) Oxygraph measurement of cellular mitochondrial respiration in igWAT of wt and miR-155−/−littermates at 12–16 weeks of age. Data are represented as means±s.e.m. (*P<0.05; Student’st-test; wt groupn=6, miR-155−/−groupn=5). Figure 6: miR-155 regulates cold-induced thermogenesis in BAT and ‘browning’ of WAT. ( a ) Representative infrared thermographic image of 12–16-week-old male wt and miR-155 −/− littermates kept at 4 °C for 4 h. ( b ) Statistical analysis of body surface temperature as measured by infrared thermography. Data are represented as means±s.e.m. (*** P <0.001; Student’s t -test; n.s., not significant; wt group n =7, miR-155 −/− group n =5). ( c ) Hematoxylin and eosin staining of interscapular BAT sections from wt and miR-155 −/− littermates kept at room tempertaure (RT) or post cold exposure (4 °C, 4 h). Scale bar, 50 μm. ( d ) Lipolysis assay of BAT from 12-week-old wt and miR-155 −/− littermates kept in 4 °C for 4 h. Data are represented as means±s.e.m. (* P <0.05; Student’s t -test; n =4). ( e ) Ex vivo oxygraph measurement of cellular mitochondrial respiration in BAT 12–16-weeks-old wt or miR-155 −/− littermates exposed to 4 °C. Data are represented as means±s.e.m. (* P <0.05; Student’s t -test; wt group n =6, miR-155 −/− group n =5). ( f ) qRT–PCR analyses of UCP1 and PGC-1α expression in BAT of 12–16-week-old wt or miR-155 −/− littermates after cold exposure. Data are represented as means±s.e.m. (* P <0.05; Student’s t -test; n =4). ( g ) Representative hematoxylin and eosin staining of igWAT sections from wt and miR-155 −/− littermates at RT or post cold exposure (top). Immunohistochemical staining for UCP1 abundance in respective igWAT sections (bottom). Scale bar, 50 μm. ( h ) qRT–PCR analyses of UCP1 and PGC-1α in igWAT 12–16-week-old wt or miR-155 −/− littermates exposed to 4 °C for 4 h. Data are represented as means±s.e.m. (* P <0.05; Student’s t -test; wt group n =4, miR-155 −/− group n =4). ( i ) Oxygraph measurement of cellular mitochondrial respiration in igWAT of wt and miR-155 −/− littermates at 12–16 weeks of age. Data are represented as means±s.e.m. (* P <0.05; Student’s t -test; wt group n =6, miR-155 −/− group n =5). Full size image Analysis of BAT morphology revealed fewer lipid droplets in miR-155 −/− mice after 4 °C treatment ( Fig. 6c ). Exposure to cold increased lipolytic activity and cellular respiration to a greater extent in miR-155 −/− mice than in wt mice ( Fig. 6d ), which could explain the reduced lipid content of miR-155 −/− BAT. Moreover, miR-155 −/− mice exhibited increased expression of UCP1 and PGC-1α ( Fig. 6f ). Given the impact of miR-155 on the development of a brown fat-like thermogenic program in white adipocytes (see also Fig. 5d ), we studied whether cold-induced WAT browning is affected by loss of miR-155 in vivo. igWAT of miR-155 −/− mice kept at ambient temperature was clearly morphologically different from wt mice ( Fig. 6g ) and contained clusters of brown-like, multilocular adipocytes ( Fig. 6g ). After cold exposure, the induction of a brown fat phenotype in WAT was clearly enhanced in miR-155 −/− mice with the predominant small, multilocular adipocytes. Furthermore, we found a stronger induction of UCP1 and PGC-1α expression, and enhanced cellular respiration in miR-155 −/− mice compared with wt littermates ( Fig. 6g–i ). Body weight of 12–16-week-old miR-155 −/− mice was significantly lower, whereas food intake of these animals was not altered when compared with wt littermates ( Supplementary Fig. S8a,b ). Importantly, we found that even heterozygous miR-155 (miR-155 +/− ) mice that express circa 50% less miR-155 than wt mice ( Supplementary Fig. S8c ) showed significantly enhanced thermogenesis and cellular respiration ( Supplementary Fig. S8d–h ). Respiration rates of both miR-155 +/− BAT and igWAT were significantly increased ( Supplementary Fig. S8g,h ). These findings show that changes of miR-155—even at moderate levels—induce activation of the thermogenic program in BAT and WAT depots. Adipocytes of interscapular BAT originate from Myf5-positive progenitors [13] . In addition, brown-like cells with multilocular morphology and UCP1 expression have been described in WAT that are not derived from Myf5-positive precursor cells [42] . The development of these beige cells is induced by cold-exposure or β 3 -agonist treatment [43] . Other stimuli that enhance recruitment of beige cells include prostaglandins, the transcription factor FOXC2 and PPARγ agonists (thiazolidinediones) [4] , [44] , as well as natriuretic peptides and cyclic guanosine monophosphate [45] , [46] . So far, not much was known about miRNA-based regulation of brown and beige adipocytes. miRNAs control the expression of a large part of the human and murine genome. Initial studies revealed differential expression of miRNAs in white and brown adipocytes and expression of muscle-specific miRNAs in brown adipocytes [11] . A recent study [12] found that miR-193b-365 cluster enhances in vitro brown adipogenesis. Using deep sequencing, we identified miRNAs that are differentially expressed during brown adipogenesis. Among these miRNAs, miR-155 was of special interest as it efficiently inhibited adipogenesis and was enriched in BAT. Moreover, C/EBPβ, a crucial pro-adipogenic transcription factor, had been identified as a major miR-155 target in other cell types including white preadipocytes [21] , [22] , [23] . Brown and white fat differentiation share many transcriptional regulators [47] . For example, PPARγ has been identified as a master regulator of both white and brown adipogenesis. In contrast, there appears to be a specificity of certain C/EBPs for white versus brown fat. C/EBPα is required for differentiation of WAT, but not BAT [48] . The analysis of C/EBPβ and C/EBPβ-/C/EBPδ-knockout mice revealed a predominant role of C/EBPβ in BAT [16] , with only little effects in white fat. This preferential effect of C/EBPβ in BAT might be explained by (i) differences in the temporal dynamics of C/EBPβ expression, with sustained C/EBPβ exposure resulting in a brown phenotype [49] and/or (ii) by its interaction with the transcriptional coregulator PRDM16. PRDM16 and C/EBPβ are co-enriched in BAT and form a transcriptional complex that controls the cell fate switch to brown fat cells [18] , [43] . Interestingly, overexpression of C/EBPβ alone induces a brown fat cell-like phenotype in white adipocytes [49] . The correct timing of C/EBPβ expression is crucial for adipogenic differentiation. An intricate network of regulators controls C/EBPβ expression and function. Among these are adipogenic hormones like insulin, transcription factors (for example, CREB, Hoxc8 and Plac8), as well as post-transcriptional regulators (for example, KSR1 and TRB3) [17] , [50] , [51] , [52] , [53] . miR-155-based post-transcriptional regulation adds another level of regulation. miR-155 shows an interesting temporal expression pattern with high levels during preadipocyte proliferation and decreasing expression during maturation. Similar regulatory patterns have been described for Plac8 (ref. 17 ). Overall, miR-155 can be classified as a miRNA inhibitor of brown fat adipogenesis. Similar to the situation in cancer, where tumour promoting, oncogenic miRNAs and tumour-suppressive, anti-oncogenic miRNAs have been identified [7] , we propose that an interplay of ‘pro-adipogenic’ miRNAs—such as miR-193b-365 and miR-196a [12] , [53] —and ‘anti-adipogenic’ miRNAs like miR-155 orchestrate adipogenic differentiation. Importantly, we found a reciprocal negative regulation ( Fig. 7 ) between miR-155 and C/EBPβ that integrates pro- and anti-adipogenic cues. One such anti-adipogenic cue is TGFβ1, which is secreted by proliferating preadipocytes and induces miR-155 expression. High levels of miR-155 inhibit C/EBPβ expression, thereby suppressing premature differentiation and keeping preadipocytes in an undifferentiated state. Pro-adipogenic hormones induce expression of C/EBPβ, which in turn inhibits transcription of BIC/miR-155. Thereby, this double-negative feedback mechanism leads to robust commitment to one of the two possible states establishing a bistable system [36] . A similar bistable system has been described for miR-7 and the transcription factor Yan in the developing Drosophila eye [54] . The miR-155/C/EBPβ bistable loop might have evolved to convert weak or only transiently available external signals to a strong response, ensuring a uniform response of precursor cells to signals that either prohibit or induce adipogenesis. 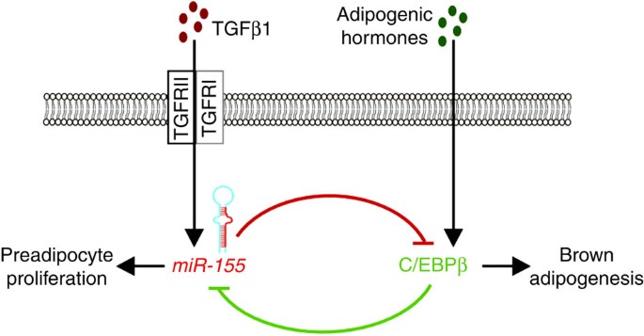Figure 7: Schematic model of miR-155-regulated brown adipogenesis. miR-155 and C/EBPβ form a self-inhibitory feedback loop that tightly regulates brown adipogenesis. miR-155 expression is induced by TGFβ1 signalling and mediates translational repression of C/EBPβ by binding to its 3′ UTR. In turn, C/EBPβ is induced by adipogenic hormones and inhibits transcription of miR-155. Thereby, miR-155 and C/EBPβ constitute a bistable system for the regulation of adipogenesis and thermogenesis by either maintaining preadipocytes in an undifferentiated precursor state (mitotic clonal expansion) or initiating the brown adipogenic program. Figure 7: Schematic model of miR-155-regulated brown adipogenesis. miR-155 and C/EBPβ form a self-inhibitory feedback loop that tightly regulates brown adipogenesis. miR-155 expression is induced by TGFβ1 signalling and mediates translational repression of C/EBPβ by binding to its 3′ UTR. In turn, C/EBPβ is induced by adipogenic hormones and inhibits transcription of miR-155. Thereby, miR-155 and C/EBPβ constitute a bistable system for the regulation of adipogenesis and thermogenesis by either maintaining preadipocytes in an undifferentiated precursor state (mitotic clonal expansion) or initiating the brown adipogenic program. Full size image To gain further insight into the function of miR-155, we generated miR-155 transgenic mice. These transgenic animals showed reduced BAT mass, altered BAT morphology and significantly reduced UCP1 expression. This phenotype corresponds to the impaired differentiation of miR-155-overexpressing preadipocytes observed in vitro . Interestingly, the level of miR-155 overexpression achieved in the miR155TG mice caused only a slight—albeit significant—reduction of C/EBPβ, indicating that the major effect of miR-155 transgenesis is not a mere suppression of C/EBPβ but rather a destabilization of the miR-155-C/EBPβ feedback loop tipping the balance towards an undifferentiated state. In line with reduced brown fat differentiation and reduced UCP1 levels, we found significantly reduced BAT thermogenesis in miR-155 transgenic mice. BAT-specific expression of miR-155 using the UCP1 promoter resulted in the same effects, indicating that the observed phenotype is cell autonomous. Concerning the effect of miR-155 on WAT, the in vitro data show that miR-155 expressed at high levels can inhibit differentiation of murine WAT, human MSCs [23] and 3T3-L1 cells [24] . In contrast to BAT, we found no significant changes in WAT weight in the miR-155 transgenic mice, although both tissues expressed similar levels of miR-155. Overall, the phenotype of miR-155 transgenics strikingly resembles C/EBPβ −/− mice [16] . Our in vivo studies included acute exposure (to 4 °C for 4 h) of miR-155 −/− mice. This test mainly examines cold tolerance, which is determined by BAT-derived thermogenesis, as well as muscle-derived shivering and cold-stress [55] . The cold-exposure data provide clear evidence for increased BAT function in the absence of miR-155: the drop in body temperature is significantly reduced in cold-exposed miR-155 −/− mice. Importantly, miR-155 −/− mice show dramatic morphological changes in BAT after 4 h cold exposure in comparison with wt animals with a strong decrease of the number and size of lipid droplets. In addition, they have increased levels of UCP1 and PGC-1α. Finally, BAT dissected from miR-155 −/− animals post cold exposure displays significantly higher levels of glycerol release and cellular respiration. Our study also unravels a decisive function of miR-155 in controlling ‘browning’ of white fat: miR-155 depletion activates the thermogenic program in white adipocytes. Consequently, miR-155 −/− mice show an increased ability to adapt to cold exposure and recruit inducible brown/beige cells. Thus, miR-155 is a key regulator of brown adipocyte identity in brown as well as in white fat. Concerning a potential role of miR-155 in humans, it is of interest that miR-155 expression has been associated with adipose tissue dysfunction and obesity [56] . Because reduction of miR-155 by 50% in mice already enhances recruitment of brite fat cells and differentiation of BAT, therapeutic attempts to reduce miR-155 might be a promising approach to treat obesity in humans. Animal studies with miR-155 transgenic and miR-155 −/− mice To obtain miR-155 transgenic mice, a PGK or UCP1 promoter-driven eGFP mRNA/pre-miR-155 cassette was cloned into a lentiviral vector. High-titre virus was used to transduce preimplantation embryos as described previously [38] . Genotypes were assessed by PCR detection of the eGFP cassette in genomic DNA. miR-155 −/− C57BL/6J mice were purchased from Jackson laboratory. For cold-exposure experiments, 12–16-week-old male mice were exposed to 4 °C for 4 h. The study was approved by the Landesamt für Natur, Umwelt und Verbraucherschutz Nordrhein-Westfalen, Germany. Primary preadipocyte culture and differentiation Interscapular BAT cells were isolated from newborn pups [20] , and igWAT cells were isolated from 10–12-week-old C57BL/6J mice. After digestion with collagenase and centrifugation, preadipocytes/SVF were seeded in six-well plates with DMEM supplemented with 10% fetal bovine serum, and 1% Pen/Strep (day −4). For BAT in vitro differentiation, the cells were treated with differentiation medium containing 20 nM insulin and 1 nM triiodothyronine (T3) from day −2 to day 0 and induced with induction medium supplemented with 20 nM insulin, 1 nM T3, 0.5 mM isobutylmethylxanthine and 1 μM dexamethasone from day 0 to day 2. Differentiating cells were kept in differentiation medium from day 2 to day 8 ( Supplementary Fig. S1a ). For WAT in vitro differentiation, fully confluent cells were kept in growth medium for 2 days, then treated with induction medium supplemented with 1 μg ml −1 insulin, 1 nM T3, 0.25 μM dexamethasone, 0.5 mM isobutylmethylxanthine, 1 μM rosiglitazone and ABP (50 μg ml −1 L - A scorbate, 1 μM B iotin and 17 mM P antothenate). After 6 days, the cells were kept in medium supplemented with 1 μg ml −1 insulin, 1 nM T3 and ABP for 4 to 5 days. Medium was exchanged every 2 days ( Supplementary Fig. S7a ). Deep sequencing Deep sequencing [57] (including miRNA cloning and library sequencing) was performed by Vertis Biotech (Munich, Germany) with total RNA samples from brown preadipocytes (SVF) and in vitro differentiated mature BAT cells. Plasmids and viral infection Lentiviral vectors were constructed by cloning GFP cDNA, murine precursor miRNAs, control miRNAs, sponge miRNAs or murine C/EBPβ cDNA into the vectors p156rrlCMV and p156rrlpgk1. The control vector (p156rrl) contained no transgene (LVcontrol). Retroviral vectors carrying C/EBPβ siRNA were kindly provided by Professor Jeffrey Friedman [58] . For lentivirus production [38] , vector plasmids as well as the packaging plasmids pMDLg/pRRE, RSV-rev and pMD2.G were co-transfected into HEK 293 T cells (ATCC) seeded on Poly- L -lysine-coated 150-mm 2 dishes. Cells were incubated at 37 °C and 3% CO 2 overnight. Medium was changed 12, 48 and 72 h later. The supernatant was collected and centrifuged by an ultracentrifuge with SW32 Ti rotor at 61,700 g at 17 °C for 2 h. Combined virus suspensions were concentrated by centrifugation over a 20% (w/v) sucrose cushion in a SW55 Ti rotor at 53,500 g at 17 °C for 2 h. For functional in vitro analyses, preadipocytes were transduced with the respective virus at day −4 and then differentiated to day 8 post full confluency. Viral titer was quantified using RTase enzyme-linked immunosorbent assay. pGL3 luciferase constructs containing the BIC/miR-155 promoter were gifts from Professor E. Flemington [35] . The C/EBPβ 3′ UTR was cloned into the dual-luciferase reporter constructs pMIR-RNL-TK. pCDNA3.1-C/EBPβ, C/EBPα and C/EBPδ expression vectors were purchased from Addgene. Oil Red O staining and TG content measurement Cells were fixed in 4% paraformaldehyde for 20 min and then stained with Oil Red O solution (5 mg ml −1 in isopropyl alcohol; Sigma) for 4 h at RT. Stained cells were washed three times with water and visualized. Differentiated brown adipocytes were washed once with PBS, lysed with TX lysis buffer (150 mM NaCl, 0.05% Triton-X 100 and 10 mM Tris-HCl, pH 8) and frozen. TG reagent (Sigma) was added to thawed, homogenized lysates, and absorption (540 nm) was measured after 5 min incubation at 37 °C. The TG content was normalized to the protein content of the sample, obtained by Bradford assays. Proliferation assay Cell number was determined using the PrestoBlue Cell Viability Reagent (Invitrogen) according to the manufacturer’s instructions. Promoter analyses Computational analysis of the BIC/miR-155 promoter sequence for identification of putative transcription-factor-binding sites was performed using the TFSEARCH ver.1.3 database. Luciferase reporter assays HIB-1B brown adipose cells, kindly provided by Professor M. Klingenspor (Technical University Munich, Germany), were transiently transfected by Lipofectamine 2000 (Invitrogen) according to the manufacturer’s instructions. Cell extracts were prepared 48 h after transfection, and luciferase assays were performed using the Dual Luciferase Reporter Assay System (Promega). pGL3-BIC/miR-155 promoter assays were normalized to Renilla luciferase activity from the co-transfected pRL-TK vector (Promega). RNA isolation and qRT–PCR Total RNA was isolated from cells or tissues using Trizol (Invitrogen). Reverse transcription were performed using the Transcriptor First Strand Synthesis Kit (Roche). PCR was performed with SYBR-Green (Roche) using a HT7900 instrument (Applied Biosystems). Fold changes were calculated using relative quantification methods (ΔΔCt) with HPRT (hypoxanthine guanine phosphoribosyl transferase) serving as internal control. For miRNA expression analysis, reverse transcription of total RNA and quantitative PCRs were performed using TaqMan MIRNA Assays (Life Technologies) according to the manufacturer’s instructions. SnoRNA202 served as internal control. For primer sequences refer to Supplementary Table S1 . Western blotting Proteins from cells and tissues were extracted with RIPA lysis buffer (150 mM NaCl, 50 mM Tris-HCl, pH 7.5, 1% Nonidet P40, 0.25% Na-deoxycholate and 0.1% SDS) containing Complete protease inhibitor cocktail (Roche), 1 mM Na 3 VO 4 and 10 mM NaF. Western Blotting [20] was performed with anti-FABP4 (aP2) (1:1,000), anti-C/EBPα (1:1,000), anti-C/EBPβ (1:800), anti-UCP1 (1:500) and anti-PPARγ (1:1,000) antibodies that were purchased from Santa Cruz Biotechnology or Sigma-Aldrich. The anti-Pref-1 (1:800) antibody was purchased from Cell Signaling Technologies. Anti-β-tubulin (1:1,000) antibody was purchased from Upstate and served as loading control. Densitometric analyses were carried out using the QuantityOne software (Bio-Rad). Lipolysis assay Glycerol release from BAT tissue was measured by chopping and incubating the tissue in lipolysis medium at 37 °C and 5% CO 2 for 2 h. Glycerol release was calculated and normalized to the tissue weight, which was measured before chopping the tissue. Measurement of endogenous respiration Adipose tissue (about 3–6 mg BAT or 30–50 mg igWAT) from 12–16-week-old, cold-exposed (4 h, 4 °C) wt, miR-155 +/− or miR-155 −/− mice was isolated immediately before oxygraphic measurements (Oxygraph 2K; Oroboros Instruments). Tissue was dissected into small pieces and transferred to the oxygraph chamber containing 2 ml incubation medium (0.5 mM EGTA, 3 mM MgCl 2 ·6H 2 O, 60 mM K-lactobionate, 20 mM taurine, 10 mM KH 2 PO 4 , 20 mM HEPES, 110 mM sucrose and 1 g l −1 BSA, pH 7.1) with 25 μg ml −1 digitonin. Ex vivo respiration levels of the adipose tissues were recorded when reaching a steady state. Respiration rates were normalized to total protein content. Enzyme-linked immunosorbent assay Cell culture supernatants were collected every 2 days throughout in vitro differentiation [20] . TGFβ1 enzyme-linked immunosorbent assays were performed according to the manufacturer’s instructions (R&D Systems). Chromatin immunoprecipitation wt primary brown preadipocytes were transduced with LVC/EBPβ or LVcontrol. ChIP assay was performed following the manufacturer’s instructions (Agarose ChIP kit; Pierce). Anti-C/EBPβ antibody (1:35) (Santa Cruz Biotechnology) was used to precipitate C/EBPβ-bound DNA. qRT–PCR analysis on recovered DNA fragments was performed using primers that span the putative C/EBPβ-binding sites A, B/C/D or E, respectively ( Supplementary Table S1 ). qRT–PCR results were normalized to input values. Histology and microscopy Adipose tissue was fixed in 4% paraformaldehyde in PBS for 24 h at 4 °C, then paraffin-embedded. Hematoxylin and eosin staining was performed on 4 μm paraffin-embedded interscapular BAT sections and 5 μm paraffin-embedded igWAT according to the standard protocols. Immunohistochemical stainings were performed on paraffin sections, with a UCP1 antibody (1:500, rabbit anti-UCP1; Abcam), and a secondary antibody-conjugated with horseradish peroxidase (1:200, anti-rabbit; Santa Cruz Biotechnology), and visualized using DAB substrate (Vector). Nuclei were stained with hematoxylin. Statistics Values are presented as means±s.e.m. Statistical differences between two means were determined using Student’s t -test (unpaired, two-tailed), and one-way analysis of variance was used to compare differences among multiple groups. GraphPad Prism 5 or Excel software was used to calculate P -values ( * P <0.05, ** P <0.01 and *** P <0.001). Accession codes : miRNA expression have been deposited in the Gene Expression Omnibus (GEO) database under accession codes GSE45499 . How to cite this article: Chen, Y. et al . miR-155 regulates differentiation of brown and beige adipocytes via a bistable circuit. Nat. Commun. 4:1769 doi:10.1038/ncomms2742 (2013).